Considerably improved photovoltaic performance of carbon nanotube-based solar cells using metal oxide layers Carbon nanotube-based solar cells have been extensively studied from the perspective of potential application. Here we demonstrated a significant improvement of the carbon nanotube solar cells by the use of metal oxide layers for efficient carrier transport. The metal oxides also serve as an antireflection layer and an efficient carrier dopant, leading to a reduction in the loss of the incident solar light and an increase in the photocurrent, respectively. As a consequence, the photovoltaic performance of both p -single-walled carbon nanotube (SWNT)/ n -Si and n -SWNT/ p -Si heterojunction solar cells using MoO x and ZnO layers is improved, resulting in very high photovoltaic conversion efficiencies of 17.0 and 4.0%, respectively. These findings regarding the use of metal oxides as multifunctional layers suggest that metal oxide layers could improve the performance of various electronic devices based on carbon nanotubes. Over the past decade, photovoltaic devices using nanoscale materials, such as semiconductor quantum dots [1] , [2] , [3] , nanowires [4] , [5] , [6] and so on [7] , have been extensively studied. Carbon nanotubes with cylinder-like, one-dimensional structures have attracted much interest for photovoltaic applications because of their electronic and optical properties [8] , [9] , [10] , [11] , including the ability to tune their band gaps over a wide wavelength range [12] , high carrier mobilities along their one-dimensional axes [13] , [14] and high optical transparency values with low resistivity [15] . Indeed, a variety of photovoltaic devices using carbon nanotubes such as carbon nanotube-based organic solar cells [16] , photoelectrochemical cells [17] , dye-sensitized solar cells [18] and carbon nanotube/Si solar cells [19] , [20] have been reported. Furthermore, the importance of carbon nanotubes as photovoltaic materials is continually increasing. However, several crucial issues remain to be solved for further improvement of the carbon nanotube photovoltaic device performance and to enable the shift from the fundamental research to the technological applications development. First, a high Schottky barrier at the interface of the carbon nanotubes and the metal electrode limits the performance in carbon nanotube-based photovoltaic devices. Control of the Schottky barrier using an efficient carrier transport layer should enable the delivery of a high current without the carrier recombination loss [21] . Second, more efficient carrier doping for the carbon nanotubes is required to reduce the series resistance loss and increase the power conversion efficiency. Third, solar light management within the device structure of the carbon nanotube solar cells is required to enhance the photocarrier generation efficiency. In this paper, we report on the improvement in the photovoltaic performance of the carbon nanotube-based solar cells containing environmentally friendly, durable and inexpensive MoO x and ZnO metal oxide layers. The MoO x and ZnO layers play multiple roles as antireflection, carrier doping and efficient carrier transport layers in the carbon nanotube-based solar cells. The photovoltaic performance of the single-walled carbon nanotube (SWNT)/Si hybrid solar cells is improved using these multifunctional MoO x and ZnO layers, with high power conversion efficiencies (PCE) of 17.0 and 4.0% achieved for p -SWNT/ n -Si and n -SWNT/ p -Si devices, respectively. The 17.0% PCE value is the highest yet reported for the PCE of p -SWNT and the 4.0% PCE value is also quite high compared to the n -SWNT hybrid solar cells reported in the literature. The detailed physical mechanism of the multifunctional layers is also discussed. 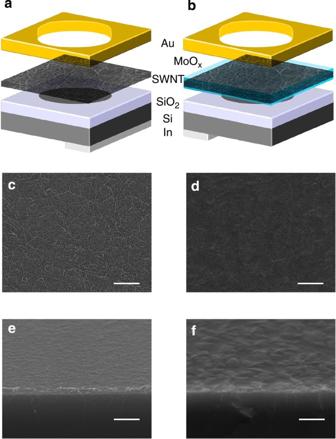Figure 1: Schematics of the solar cell devices and characterization of the SWNT network film. (a,b) Schematics of the pristine-SWNT/Si and MoOx-SWNT/Si solar cells, respectively. (c,d) Top-view SEM images of the SWNT network film on an Si wafer and the SWNT film with an MoOxlayer, respectively. (e,f) Cross-sectional SEM images of the pristine-SWNT/Si and MoOx-SWNT/Si solar cells, respectively. Scale bar in each figure is 1 μm. Structure of the solar cells Figure 1a,b shows schematics of the p -SWNT/ n -Si heterojunction solar cells without and with an MoO x layer, respectively. To fabricate the p -SWNT/ n -Si heterojunction solar cells with the MoO x layer, the MoO x layer is evaporated on the SWNT network film, and then a gold (Au) contact is coated using the mask of the active window area. The MoO x layer consists of two parts; one section of the MoO x layer is sandwiched by the SWNT film and the Au contact, and the other one is only in contact with the SWNT film in the window area of the solar cell. Figure 1: Schematics of the solar cell devices and characterization of the SWNT network film. ( a , b ) Schematics of the pristine-SWNT/Si and MoO x -SWNT/Si solar cells, respectively. ( c , d ) Top-view SEM images of the SWNT network film on an Si wafer and the SWNT film with an MoO x layer, respectively. ( e , f ) Cross-sectional SEM images of the pristine-SWNT/Si and MoO x -SWNT/Si solar cells, respectively. Scale bar in each figure is 1 μm. Full size image Figure 1c,d shows the scanning electron microscope (SEM) images of the SWNT network film without and with the MoO x coating. The average diameter of the SWNTs is determined to be 1.6 nm from the absorption spectrum of the film ( Supplementary Fig. 1 ) [22] . The SWNT film without the MoO x coating exhibits a spider web-like structure consisting of the interconnected nanotube bundles with the diameters ranging from several to tens of nanometres. The evaporation of MoO x for 60 s results in the SWNT network film being covered by a very thin MoO x layer. Figure 1e,f show cross-sectional views of the SWNT/Si layers, which are used to determine the thickness of the MoO x layer. A textured surface structure is observed for the SWNT/Si with the MoO x layer ( Fig. 1f ), and the average thickness of the MoO x layer was determined to be ~40 nm. Notably, as the deposition time increased, the MoO x layer on the SWNT film becomes flat. SEM images of SWNT films coated with thicker MoO x layers are shown in Supplementary Fig. 2 . Performance of carbon nanotube solar cells with MoO x layers The current density–voltage ( J – V ) characteristics of the p -SWNT/ n -Si solar cells under the air mass (AM) 1.5 conditions are shown in Fig. 2a . Typical photovoltaic behaviour is observed; the J – V curve of the pristine-SWNT/Si solar cell (black solid line) exhibits a short-circuit current density ( J sc ) of 27.9 mA cm −2 , an open-circuit voltage ( V oc ) of 0.57 V and a fill factor (FF) of 69%, resulting in a PCE ( η ) of 11.1%. In contrast, the J – V curve for the solar cell containing the MoO x -coated SWNT film (MoO x -SWNT/Si) exhibits a very high J sc value of 36.6 mA cm −2 , which is close to the maximum value reported for Si solar cells [23] and is the highest short-circuit current density for hybrid solar cells using crystalline Si and other nanomaterials. This short-circuit current density value is associated with a V oc of 0.59 V and an FF of 78%, resulting in a very high 17.0% η value that represents a 50% increase in the PCE compared with that of the pristine-SWNT/Si solar cell. It should be noted that the thickness of the MoO x layer (~40 nm) is optimized for the MoO x -SWNT/Si solar cell ( Supplementary Figs 3 and 4 ). This very high η of 17.0% is the highest value reported to date for the carbon-based solar cells, including the SWNT/Si solar cells. Furthermore, the J – V curves for the p -SWNT/ n -Si solar cells in Fig. 2a are well reproduced by the fitted curves ( Supplementary Fig. 5 ) calculated using the equivalent circuit model (details are shown in Supplementary Note 1 and Supplementary Fig. 11 ). The values of the shunt resistance, series resistance and diode ideality factor are much improved for the MoO x -SWNT/Si solar cell and are shown in the Supplementary Table 1 . We also investigated the PCE variations among five solar cells fabricated with the optimized device parameters. 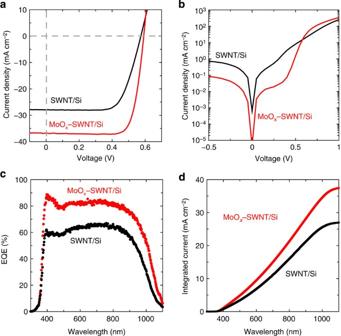Figure 2: Photovoltaic properties of the solar cell devices. (a)J–Vcurves for an SWNT/Si solar cell recorded under AM 1.5G (solid lines) and dark (dashed lines) conditions before (black lines) and after (red lines) the vapour deposition of an MoOxlayer. (b) Log-plot of the dark current before (black line) and after (red line) the deposition of the MoOxcoating. (c) IPCE spectra before (black line) and after (red line) the deposition of the MoOxcoating. (d) Calculated integrated photocurrent under AM 1.5G irradiation before (black line) and after (red line) the deposition of the MoOxcoating. A very small variation of the PCE in the 15.8–17.6% range is observed as shown in the Supplementary Table 2 . Figure 2: Photovoltaic properties of the solar cell devices. ( a ) J – V curves for an SWNT/Si solar cell recorded under AM 1.5G (solid lines) and dark (dashed lines) conditions before (black lines) and after (red lines) the vapour deposition of an MoO x layer. ( b ) Log-plot of the dark current before (black line) and after (red line) the deposition of the MoO x coating. ( c ) IPCE spectra before (black line) and after (red line) the deposition of the MoO x coating. ( d ) Calculated integrated photocurrent under AM 1.5G irradiation before (black line) and after (red line) the deposition of the MoO x coating. Full size image The J – V characteristics for both the pristine-SWNT/Si and MoO x -SWNT/Si solar cells clearly exhibit the diode properties. However, the MoO x -SWNT/Si solar cell showed much better diode properties with a lower reverse leakage current and three orders of magnitude higher rectification ratio compared with those of the pristine-SWNT/Si solar cell. This suggests a reduction of the series resistance and an increase in the shunt resistance with the addition of the MoO x coating in the SWNT/Si solar cell. An increase in the dark current under forward bias conditions above 0.5 V is also observed. This result indicates that the hole extraction efficiency is improved because of the MoO x coating [24] , [25] , which will be discussed below. Moreover, the diode ideality factor n (=1.08) for the MoO x -SWNT/Si solar cell is lower than that of the pristine-SWNT/Si (=1.24). Such a low value for the diode ideality factor is an indication of the efficient transport characteristics with minimum interfacial recombination in the MoO x -SWNT/Si solar cell. Next, the effects of the MoO x coating incorporation in the SWNT/Si solar cell are further investigated to understand the improvement in the photovoltaic properties. Figure 2c presents the spectra of the incident photon-to-current efficiency (IPCE) for the pristine-SWNT/Si and the MoO x -SWNT/Si solar cells. A broad and flat value of ~65% in the spectrum of the original pristine-SWNT/Si cell is observed from 400 to 900 nm, which corresponds to the wavelength range of Si light absorption and suggests that the Si substrate plays a role in the solar light absorption and photocarrier generation of the cell [26] , [27] , while the SWNT mainly works as the efficient carrier separation, collection and transport layer [27] . In contrast, the IPCE spectrum of the MoO x -SWNT/Si solar cell exhibits a large increase in the external quantum efficiency (EQE) and surpassed 80% for the wavelengths between 400 and 900 nm. Figure 2d shows the integrated currents calculated using the overlap between the EQE spectrum and the AM 1.5G solar photon flux for each cell. The calculated integrated photocurrent yields current densities of 27 and 36.5 mA cm −2 for the pristine-SWNT/Si and MoO x -SWNT/Si solar cells, respectively. Notably, these results are consistent with the photocurrent densities determined from the J – V curves, as shown in Fig. 2a . Roles of MoO x layer in SWNT/Si solar cells Thus, a dramatic improvement in the photovoltaic performance of the SWNT/Si solar cell due to the inclusion of an MoO x -coated SWNT film is demonstrated. The MoO x layer inserted between the SWNT film and the Au anode serves as an effective hole transporting layer. Moreover, the MoO x layer on the SWNT network film in the active window functions as an antireflection layer for the solar light and as a carrier dopant for the SWNTs. A detailed analysis of the physical mechanisms involved in the improved photovoltaic performance of the MoO x -coated SWNT film is presented below. Some materials inserted between the semiconducting hole generation layers and the anodes can increase the hole extraction/injection efficiency for optoelectronic devices through the reduction of the Schottky barrier at the interface. The semiconducting SWNT film with a diameter of 1.6 nm has a bandgap of about 0.9 eV when the exciton binding energy is taken into account [28] . The work function of the SWNTs is determined to be 4.7 eV (ref. 29 ). Because of the difference in the work functions of the SWNTs and Au (5.3 eV) [30] , an interface dipole layer is formed at the SWNT/Au-anode interface until the valence band edge of the SWNTs aligns with the Fermi level of the Au anode; this is accompanied by large band bending, as shown in Fig. 3a . Such a pinning effect involved in the alignment of the valence band edge and the Fermi level has been observed using scanning tunnelling spectroscopy [30] . The presence of the MoO x coating and the interaction between the MoO x layer and the SWNT film leads to significant changes in the electronic structure of the SWNT surface and the consequent modification of the surface potential. The work function of the MoO x layer is higher than the ionization energy of the SWNTs and is close to the Fermi level of the SWNTs; this enables efficient hole transfer from the SWNTs to the Au anode via the MoO x layer. MoO x films have been frequently observed to function as hole transport layers in organic semiconductor/Au interfaces [31] . The change in the band alignment due to the insertion of the MoO x layer promotes photocarrier extraction from the SWNTs to the Au anode, leading to a significant increase in the short-circuit current density and a reduction of the net series resistance ( R s ) value. Therefore, as an effective hole transport layer, MoO x enhances the photovoltaic performance by preventing current leakage and consequent counter-diode formation [32] , as is also illustrated in Fig. 2b . 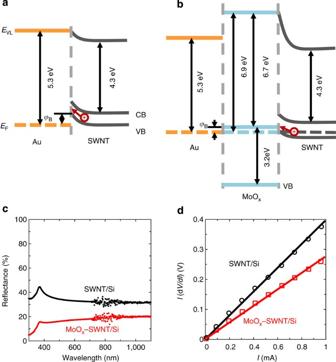Figure 3: Multifunctional performance of MoOxlayer. (a,b) Bandgap alignments of the pristine-SWNT/Au and the MoOx-SWNT/Au interfaces, respectively. (c) Reflectance spectra of the pristine-SWNT/Si (black line) and MoOx-SWNT/Si (solid line) solar cells. (d)I(dV/dI) plots of the pristine-SWNT/Si (black line) and MoOx-SWNT/Si (red line) solar cells as a function of the currentI. Figure 3: Multifunctional performance of MoO x layer. ( a , b ) Bandgap alignments of the pristine-SWNT/Au and the MoO x -SWNT/Au interfaces, respectively. ( c ) Reflectance spectra of the pristine-SWNT/Si (black line) and MoO x -SWNT/Si (solid line) solar cells. ( d ) I (d V /d I ) plots of the pristine-SWNT/Si (black line) and MoO x -SWNT/Si (red line) solar cells as a function of the current I . Full size image To reveal the role of the MoO x film as a hole transport layer, a p -SWNT/ n -Si solar cell with an MoO x layer between the SWNT film and the Au anode is fabricated ( Supplementary Fig. 6 ). The η value of 14.2% for the p -SWNT/ n -Si solar cell with the MoO x coating on the active area is much enhanced compared with η= 11.5% obtained for the pristine-SWNTs/Si solar cell. On the basis of this result, it is concluded that the PCE value increases because the MoO x layer acts mainly as a hole extraction layer and reduces the Schottky barrier height at the interface between the SWNT film and the Au anode. Next the reflectance spectra of the pristine-SWNT/Si and MoO x -SWNT/Si solar cells are obtained to evaluate the ability of the MoO x layer to act as the antireflection layer, as shown in Fig. 3c . The reflectivity ( R ) of the pristine-SWNT/Si solar cell is ~30%, mainly because of the high refractive index of Si for wavelength between 400 and 1,000 nm. On the other hand, the reflectivity of the MoO x -SWNT/Si solar cell is substantially lower over the entire spectral region from 300 to 1,100 nm (<20%). This decrease in the reflectivity contributes to the increase in the solar light absorption and the generation of the photocarriers in the Si substrate, resulting in an enhancement of the short-circuit current density. This assumption is confirmed by the evaluation of the internal quantum efficiency (IQE) using the relationship IQE=EQE/(1− R ) ( Supplementary Note 2 ). The calculated IQE spectrum of the MoO x -SWNT/Si solar cell is nearly coincident with that of the pristine-SWNT/Si, which strongly suggests that a reduction in the reflectivity contributes to the increased EQE in the MoO x -SWNT/Si solar cell ( Supplementary Fig. 8 ). The MoO x layer reduced the effective refractive index mismatch between Si and air, because MoO x has an intermediate refractive index ( n 0 =2.2) [33] . This decrease in the reflectivity of the MoO x -SWNT/Si solar cell reduced the loss of solar light and increased photocarrier generation and was due to the fact that the MoO x layer acts as an antireflection layer. The MoO x also plays a role as a carrier dopant for the SWNTs. Figure 3d shows the I (d V /d I ) plots for the pristine-SWNT/Si and MoO x -SWNT/Si solar cells as a function of the current ( I ). The R s of the solar cells without and with the MoO x coating is evaluated from the slope of this plot, and the resistance of the MoO x -SWNT/Si solar cell (=244 Ω) is found to be significantly lower than that of the pristine-SWNT/Si (=360 Ω). The decrease of the R s is also confirmed by the independent two-probe method ( Supplementary Fig. 10 , Supplementary Table 3 and Supplementary Note 3 ). Hole doping for the SWNTs in the MoO x -SWNT occurs because the ionization energy of SWNTs is lower than the work function of the MoO x layer, and thus the series resistance decreased [34] . We also confirm the effect of hole doping for SWNTs by the MoO x layer using Raman spectra ( Supplementary Fig. 9 ), which are similar to the previously reported results [34] . Therefore, an SWNT/Si solar cell with an MoO x layer only on the active window ( Supplementary Fig. 7 ) was fabricated to evaluate the antireflection layer and hole doping effects of the MoO x layer. On the basis of the J – V curves obtained for this MoO x -SWNT/Si solar cell, the value of J sc is found to be increased by ~6.5 mA cm −2 in the MoO x -SWNT/Si solar cell compared with that of the cell without the metal oxide layer. Furthermore, in the IQE spectra, an increase in the IQE is also observed for the cell with the MoO x layer, indicating the effective hole doping achieved by the addition of the MoO x coating. We quantitatively evaluated the contribution of the MoO x coating to the PCE increase ( Supplementary Note 4 ). The possibility of surface passivation by the MoO x coating was also checked ( Supplementary Fig. 12 ) [35] , [36] . However, we could not observe these effects. The increased PCE by the MoO x coating is estimated to arise from the changes in the series resistance, shunt resistance and diode loss from the equivalent circuit model [26] , [37] , and the reflection loss of solar light. The series resistance including the components of the SWNT film sheet resistance and the contact resistance for the SWNT/Au interface drastically decreases from 360 (2.83) to 117 Ω (0.92 Ω cm 2 ), resulting in the PCE improvement of 2.08%. Further, PCE increase of 1.46 and 0.09% are due to the reduction of recombination loss and diode loss, respectively, resulted due to an increase in the shunt resistance. Moreover, the estimated reduction of the reflected solar light by the antireflection effect increase the current density by 5.9 mA cm −2 ( Supplementary Note 2 ), resulting in the PCE improvement of 2.25%. The evaluated total increase of 5.9% is good agreement with the experimentally observed PCE improvement due to the MoO x coating, as shown in Fig. 2a . These quantitative results strongly support the hypothesis that the MoO x acts as a dopant and hole transporting layer, and as an antireflection layer, drastically improving the photovoltaic performance of the SWNT/Si solar cells. A statistic distribution of photovoltaic characteristics is shown in Supplementary Fig. 13 . The high value of conversion efficiencies and small distribution of SWNT/MoO x /Si solar cells show a high reproducibility of the photovoltaic devices. n -SWNT/ p -Si solar cells with ZnO layer Finally, to determine if a similar improvement in photovoltaic performance could be achieved for a cell based on the n -type carbon nanotubes, similar experiments were performed using an n -SWNT/ p -Si solar cell with ZnO insertion layers. In this study, n -SWNT/ p -Si solar cells with and without a ZnO layer between the SWNT network film and the electrode were fabricated. Details of the fabrication procedure are provided in the Supplementary Note 5 and the morphology of the ZnO layer is shown in Supplementary Fig. 15 . 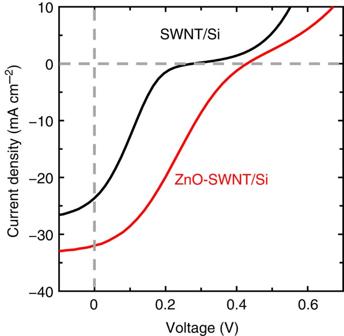Figure 4: Photovoltaic performance ofn-SWNT/p-Si solar cells. J–Vcurves for then-SWNT/p-Si solar cells without (black line) and with (red line) a ZnO layer. Figure 4 shows the J – V characteristics of the n -SWNT/ p -Si (solid black line) and ZnO-SWNT/Si (red solid line). Even for the n -SWNT/ p -Si cell without the ZnO layer, the PCE determined from the J – V curve is 1.3%. Moreover, a drastic increase in the PCE to 4.0% is observed for the ZnO-SWNT/Si cell ( Supplementary Table 4 ). The enhancement of the PCE resulted from an increase in the short-circuit current density and FF in the n -SWNT/ p -Si solar cell fabricated with the ZnO-coated SWNT film. The increased short-circuit current density results from a reduction in the loss of the solar light reflectance, an efficient extraction of the electrons to the contact and a decrease in the series resistance of the SWNTs. Moreover, the FF increases because of a reduction in the series resistance with the increase in the carrier doping ( Supplementary Fig. 14 ). These results indicated that similar to MoO x , the ZnO layer plays several roles, acting as an antireflection layer, a carrier dopant and an electron transport layer and leads to a drastic improvement in the photovoltaic performance of the n -SWNT/ p -Si solar cells. Figure 4: Photovoltaic performance of n -SWNT/ p -Si solar cells. J – V curves for the n -SWNT/ p -Si solar cells without (black line) and with (red line) a ZnO layer. Full size image In conclusion, we investigated the photovoltaic performance of the carbon nanotube-based solar cells using environmentally friendly, durable and inexpensive materials such as MoO x and ZnO that act as the antireflection layers for the increased optical absorption, carrier dopants for the reduction of the series resistance and effective carrier transport layers for the reduction of the Schottky barrier. The photovoltaic performance of the p -SWNT/ n -Si and n -SWNT/ p -Si heterojunction solar cells was improved using multifunctional layers of MoO x and ZnO, resulting in very high PCE values of 17.0 and 4.0%, respectively. We expect that metal oxides such as MoO x and ZnO will contribute to the improvement of the device performance not only for photovoltaics but also for other optoelectronics. Our finding also reveals new aspects of the device physics and the potential for optoelectronic applications based on the carbon nanotubes. Fabrication of the SWNT network films SWNTs were grown using the floating catalyst chemical vapour deposition method [22] , [38] , [39] . Carbon monoxide (CO) was used as the carbon source, and the catalyst particles were produced via the decomposition of the ferrocene vapour. CO (100 s.c.c.m.) was passed through a temperature-controlled cartridge containing the ferrocene powder. Additional CO (300 sccm) and CO 2 (3 s.c.c.m.) were also introduced to the furnace, and the growth temperature was set at 850 °C. The SWNT film was collected at room temperature on a membrane filter comprising cellulose acetate and nitrocellulose. The thickness of the SWNT film was controlled by varying the collection time. Device fabrication An n -Si substrate (1–10 Ω cm) was used for the solar cell devices. The native SiO 2 layer of the active window was removed using a buffered HF solution. The membrane filter with the SWNT network film was then placed on the Si substrate such that the SWNT network film was in direct contact with the top surface of the substrate. A fibre wiper was then applied to the surface of the substrate with adequate pressure to release the film from the membrane filter and create a connection between the film and the substrate. It was essential to place a drop of ethanol on the surface to ensure good contact between the film and the substrate and to densify the SWNT film [17] . The MoO x films were deposited via thermal evaporation of MoO 3 at a rate of 0.5 nm s −1 and base pressure of 5 × 10 −6 Torr. SWNT films with window sizes (φ: diameter) of 1.0 mm were used. Each SWNT film was then connected to the Au anode, while each n -Si substrate was connected to an indium (In) cathode. Characterization and measurements The optical absorption and reflectance spectra of the SWNT network films were obtained using a UV/Vis/NIR spectrophotometer (Hitachi U-4100). To perform the photovoltaic testing, the devices were irradiated using a solar simulator (San-Ei Electric XES-40S1) at AM 1.5 (~ 100 mW cm −2 ), and the current density–voltage data were recorded using a source meter (Keithley 2400). The AM 1.5 condition for the solar simulator was confirmed using a standard cell (BS-500BK). For the IPCE measurements, the devices were tested using a monochromatic Xenon arc light system (Zolix LSP-X150). The microstructure of SWNT films and the cross-sectional structures of the devices were characterized using a SEM (SEM, JEOL JEM-6500F). How to cite this article: Wang, F. et al . Considerably improved photovoltaic performance of carbon nanotube-based solar cells using metal oxide layers. Nat. Commun. 6:6305 doi: 10.1038/ncomms7305 (2015).